Ultrafast angular momentum transfer in multisublattice ferrimagnets Femtosecond laser pulses can be used to induce ultrafast changes of the magnetization in magnetic materials. However, one of the unsolved questions is that of conservation of the total angular momentum during the ultrafast demagnetization. Here we report the ultrafast transfer of angular momentum during the first hundred femtoseconds in ferrimagnetic Co 0.8 Gd 0.2 and Co 0.74 Tb 0.26 films. Using time-resolved X-ray magnetic circular dichroism allowed for time-resolved determination of spin and orbital momenta for each element. We report an ultrafast quenching of the magnetocrystalline anisotropy and show that at early times the demagnetization in ferrimagnetic alloys is driven by the local transfer of angular momenta between the two exchange-coupled sublattices while the total angular momentum stays constant. In Co 0.74 Tb 0.26 we have observed a transfer of the total angular momentum to an external bath, which is delayed by ~150 fs. The mechanism of ultrafast quenching of the magnetization triggered by a femtosecond laser pulse is currently still hotly debated. Despite the large amount of work devoted to the characterization of femtosecond demagnetization in various metallic systems [1] , [2] , [3] , [4] , [5] , [6] , [7] , [8] , [9] , [10] , [11] , so far no consensus over the sub-picosecond demagnetization mechanisms has emerged. The basic phenomena involved, especially regarding the dissipation of angular momenta, are still disputed [2] , [3] , [4] , [5] , [6] , [7] , [8] , [9] , [12] . Different other aspects are still discussed controversially, especially the timescales characterizing energy and angular momentum transfer between various degrees of freedom, such as electrons (e), spins (s) and phonons (ph). However, the literature documents critical differences between rare earth (RE) elements [4] and transition metals (TMs) [3] , [5] , [7] , [8] , [10] , [11] . The disparities lie in the couplings between e, s, and ph, and are related to the localization and hybridization of the electron orbitals carrying the spin momentum. As the loss of magnetization requires transfer of energy into the spin system and of angular momentum out of it, one of the important and unsolved questions is related to the description of the fundamental processes involving the transfer of angular momentum out of s. In earlier work, it has been proposed that phonon- or defect-mediated spin-flip scattering [5] or electron–magnon spin-flip scattering [11] can account for the transfer of angular momentum on the femtosecond timescale but recent quantitative ab inito calculations show that the contribution of electron–phonon spin-flip scattering is too small to describe the experimental femtosecond demagnetization [13] . Alternatively, ultrafast quenching of the magnetocrystalline anisotropy (MCA) has been proposed by Boeglin et al. [10] as a new mechanism of demagnetization in TM and has been supported by microscopic theoretical work [6] . Recently, a substitute for the transfer of angular momentum during the ultrafast demagnetization has been proposed [14] , [15] , [16] involving ultrafast superdiffusive spin-polarized transport. In this process, no angular momentum transfer to the lattice is required. However, the relative weights of each pre-cited contribution to the total demagnetization process are still unclear [17] , [18] , [19] , [20] . In the case of multi-lattice magnets, the situation is more complex [21] since additional mechanisms may emerge. For instance, transfer of angular momentum between magnetic lattices has been predicted by Mentink et al. [22] and ab initio density functional theory (DFT) calculations performed by Wienholdt et al. [12] have demonstrated that the transfer of angular momentum between both sublattices is a key phenomenon to establish a transient ferromagnetic-like state in FeCoGd alloys [23] . An experimental attempt to demonstrate the efficiency of such a process has been made by Graves et al. [24] using time-resolved resonant X-ray scattering in FeCoGd alloys. However, the scenario they propose for the transfer of angular momenta strongly relies on the microscopic inhomogeneity of the sample studied and cannot be viewed as a generic mechanism. Here, we report experimental results evidencing the initial conservation and the following dissipation of the total angular momentum during the demagnetization time by measuring the angular momentum in a quantitative way in ferrimagnetic TM–RE alloys. We have used time-resolved X-ray magnetic circular dichroism (XMCD) at the TM L 2,3 and RE M 4,5 edges at the BESSY II femtoslicing source of the Helmholtz-Zentrum Berlin [7] . This tool combines element, spin and orbital sensitivity [9] , [25] , [26] with femtosecond time resolution resolving the ultrafast dynamics of the orbital ( L i ( t )), spin ( S i ( t )) and total angular momentum ( J i ( t )) (where i stands for Co, Gd or Tb) in ferrimagnetic Co 0.8 Gd 0.2 and Co 0.74 Tb 0.26 alloys. Our results show on what timescales and through which microscopic mechanism the total angular momentum is conserved in the case of a multisublattice magnet. They reveal that, to conserve the total angular momentum, the ferrimagnetic system involves two compensating angular momenta that flow in opposite directions, allowing for the loss of magnetization in each subsystem during the first 140±60 fs of demagnetization and resulting in a net loss of the magnetization in the system. We have determined at what delay after the laser excitation the systems start to transfer angular momentum to the external reservoir. Backed by the ultrafast dynamics of the ratio L Co ( t )/ S Co ( t ), our results reveal an ultrafast quenching of the MCA in both ferrimagnetic films [10] . Finally, we show that the atomic description is still valid for Gd in the first hundred femtoseconds after the laser excitation, because the orbital momentum L Gd ( t )=0 at all times. Experimental details The magnetic configuration at the thermodynamic equilibrium of the two different ferrimagnetic alloy films Co 0.8 Gd 0.2 and Co 0.74 Tb 0.26 have been analysed by XMCD measurements; see Methods. Thanks to the chemical sensitivity of XMCD, our previous static measurements [27] are used to quantify the ultrafast dynamics of the angular momenta S z i ( t ), L z i ( t ) and J z i ( t ) in Co and in the RE elements. To test the possible ultrafast increase in L i ( t ) starting from an initial value L i ( t <0)=0, we study one of the most convenient cases, Gd in Co 0.8 Gd 0.2 . In contrast, the RE Tb has a large orbital momentum ( L =3) and is therefore well suited to study the demagnetization dynamics of the orbital momenta [27] . According to element-resolved hysteresis loops obtained for both alloys [27] , we conclude that our films are homogenous and are fully saturated under the applied magnetic field of 5 kOe. Therefore, we have L ( t )~ L z ( t ) and S ( t )~ S z ( t ) for Co, Gd and Tb. Thus, L ( t ) and S ( t ) are aligned parallel, so that we may define the time-dependent angular momentum J i ( t )= L i ( t )+ S i ( t ) per element i . The X-ray transmission experiment, using an infrared laser pump and X-ray probe configuration, is schematically shown in Fig. 1 . The external magnetic field is applied along the propagation direction of the X-rays. The lower part sketches the time evolution of the pump-induced atomic demagnetization on the exchange-coupled Co and RE in the multisublattice ferrimagnet. The time t 0 =0 is defined by the temporal overlap between the laser pulse and the X-ray pulse. A film thickness of 15 nm ensures a homogenous infrared laser excitation. The incident X-rays are circularly polarized and time-resolved XMCD is measured using the difference of intensities measured in transmission between two opposite magnetic fields + H and − H applied parallel to the X-rays (see Methods). 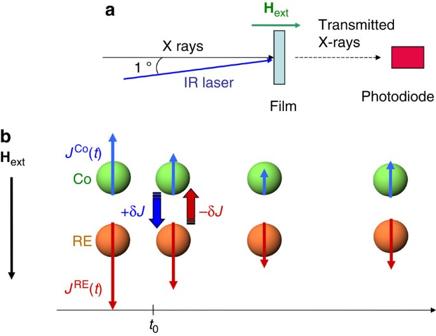Figure 1: Experimental set-up and the microscopic model. (a) Scheme of the X-ray transmission experiment using an infrared laser pump and X-ray probe configuration. The external magnetic field is applied parallel to the incoming X-rays. (b) Sketch of the time evolution of the pump-induced atomic magnetization dynamics on the exchange-coupled Co and RE in the ferrimagnetic multisublattice. Ultrafast dynamics ofJi(t) for each element is illustrated and start at the temporal overlapt0=0. At any time, both elements are exchange coupled and show antiferromagnetic order, attesting that we do not cross the compensation temperatureTcomp. During the demagnetization, a coupling between the two angular momenta may exist in the ferrimagnet. Figure 1: Experimental set-up and the microscopic model. ( a ) Scheme of the X-ray transmission experiment using an infrared laser pump and X-ray probe configuration. The external magnetic field is applied parallel to the incoming X-rays. ( b ) Sketch of the time evolution of the pump-induced atomic magnetization dynamics on the exchange-coupled Co and RE in the ferrimagnetic multisublattice. Ultrafast dynamics of J i ( t ) for each element is illustrated and start at the temporal overlap t 0 =0. At any time, both elements are exchange coupled and show antiferromagnetic order, attesting that we do not cross the compensation temperature T comp . During the demagnetization, a coupling between the two angular momenta may exist in the ferrimagnet. Full size image Ultrafast demagnetization in CoGd In Fig. 2a we show the pump-probe results obtained at the Co L 2,3 and Gd M 4,5 edges for the Co 0.8 Gd 0.2 alloy film. The normalized XMCD values at negative time delays match the XMCD magnitudes recorded at the Co L 3 , Co L 2 , Gd M 5 and Gd M 4 edges during quantitative static XMCD measurements [27] . Applying the sum rules for the Co L 2,3 and for the Gd M 4,5 edges [9] , [25] , [26] , we extract the ultrafast dynamics of the spin momentum S i ( t ) (black circles) and the orbital momentum L i ( t ) (red circles) for Co and for Gd. Quantitative data for the time-dependent values of S i ( t ) and L i ( t ) are displayed in units of ħ per atom in Fig. 2b,c (red and black symbols). The values at negative delays are normalized to the values measured at thermodynamic equilibrium [27] . The continuous lines are the results of the simulations of S i ( t ) (black line) and L i ( t ) (blue line; see Methods), whereas the green line is the ratio of these results. 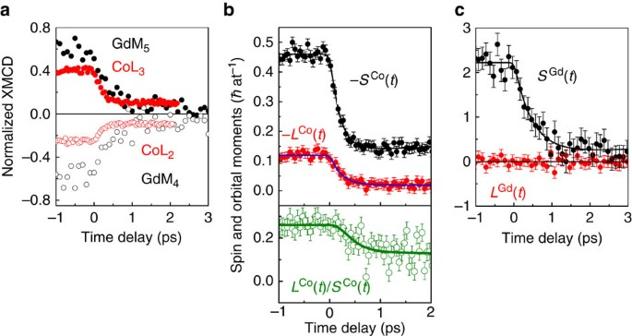Figure 2: Dynamics of spin and orbital momenta for Co and Gd in Co0,8Gd0.2. (a) Time-resolved XMCD at the Co L3(filled red circles), Co L2(empty red circles), Gd M5(filled black circles) and Gd M4edges (empty black circles) measured on a 15-nm Co0,8Gd0.2alloy film. The XMCD values at negative time delays match the XMCD magnitude recorded at the Co L3, Co L2, Gd M5and Gd M4edges during quantitative static XMCD measurements27. The pump fluence used during our experiment was adjusted to 8 mJ cm−2. (b) Ultrafast dynamics of the spin and orbital momenta −SCo(t) (black circles) and −LCo(t) (red circles) for Co as extracted by applying the sum rules. The values ofLCo(t) andSCo(t) at negative delays are normalized to the static valuesLCoandSCoat thermodynamic equilibrium27. The continuous lines are the simulations ofSCo(t) (black line) andLCo(t) (blue line; see Methods) with characteristic thermalization times ofτCotherm=200±20 fs for both momenta. The ratioLCo(t)/SCo(t) (green circle) obtained as a function of the delay time shows that the orbital momentum reduces more than the spin momentum during the ultrafast demagnetization. (c) Ultrafast dynamics of the spin and orbital momentaSGd(t) (black circles) andLGd(t) (red circles) for Gd. The values at negative delays are normalized to the static values ofLGdandSGdprovided by the static XMCD measurements27. A constant value ofLGd(t)=0 is evidenced during the ultrafast demagnetization process. The continuous line is a simulation ofSGd(t) (black line) with a characteristic thermalization time ofτGdtherm=480±40 fs. The simulations ofLi(t) andSi(t) (whereistands for Co, Gd or Tb) have been obtained using a nonlinear least square fitting procedure. The extracted error bar onτithermis the s.d., which is given as an output parameter of the fitting procedure. The error bars obtained forLi(t) andSi(t) as shown inbandcare given by the s.d. of the experimental data with respect to the fitting functions (see Methods). Figure 2: Dynamics of spin and orbital momenta for Co and Gd in Co 0,8 Gd 0.2 . ( a ) Time-resolved XMCD at the Co L 3 (filled red circles), Co L 2 (empty red circles), Gd M 5 (filled black circles) and Gd M 4 edges (empty black circles) measured on a 15-nm Co 0,8 Gd 0.2 alloy film. The XMCD values at negative time delays match the XMCD magnitude recorded at the Co L 3 , Co L 2 , Gd M 5 and Gd M 4 edges during quantitative static XMCD measurements [27] . The pump fluence used during our experiment was adjusted to 8 mJ cm −2 . ( b ) Ultrafast dynamics of the spin and orbital momenta − S Co ( t ) (black circles) and − L Co ( t ) (red circles) for Co as extracted by applying the sum rules. The values of L Co ( t ) and S Co ( t ) at negative delays are normalized to the static values L Co and S Co at thermodynamic equilibrium [27] . The continuous lines are the simulations of S Co ( t ) (black line) and L Co ( t ) (blue line; see Methods) with characteristic thermalization times of τ Co therm =200±20 fs for both momenta. The ratio L Co ( t )/ S Co ( t ) (green circle) obtained as a function of the delay time shows that the orbital momentum reduces more than the spin momentum during the ultrafast demagnetization. ( c ) Ultrafast dynamics of the spin and orbital momenta S Gd ( t ) (black circles) and L Gd ( t ) (red circles) for Gd. The values at negative delays are normalized to the static values of L Gd and S Gd provided by the static XMCD measurements [27] . A constant value of L Gd ( t )=0 is evidenced during the ultrafast demagnetization process. The continuous line is a simulation of S Gd ( t ) (black line) with a characteristic thermalization time of τ Gd therm =480±40 fs. The simulations of L i ( t ) and S i ( t ) (where i stands for Co, Gd or Tb) have been obtained using a nonlinear least square fitting procedure. The extracted error bar on τ i therm is the s.d., which is given as an output parameter of the fitting procedure. The error bars obtained for L i ( t ) and S i ( t ) as shown in b and c are given by the s.d. of the experimental data with respect to the fitting functions (see Methods). Full size image Analysing the time-dependent spin and orbital momenta for Co ( Fig. 2b ) we observe that, similar to CoPd films [10] , the magnitude of the demagnetization observed for S Co ( t ) and L Co ( t ) are different leading to a large quenching of the ratio L Co ( t )/ S Co ( t ) before t =1 ps ( Fig. 2a , green symbols). The thermalization times of S Co ( t ) and L Co ( t ) are identical ( τ therm =200±20 fs) within the error bars. For Gd ( Fig. 2c ), we notice a large decrease of S Gd ( t ) while L Gd ( t )~0. The dynamics of S Gd ( t ) show that the thermalization time is much longer, τ th =480±40 fs (ref. 27 ). Interestingly, the value L Gd ( t )=0 stays constant over this time, although the orbital momentum was previously assumed to be an angular momentum sink to explain the loss of spin momentum on the sub-picosecond timescale. The excess of angular momentum stored in the electron orbit was assumed to be transferred to the lattice only at longer times (~1 ps) [28] . A transfer to the lattice was also proposed by Stamm et al. [7] in the case of Ni, although on the faster sub-picosecond timescale. The quantitative ultrafast dynamics of S Gd ( t ) and L Gd ( t ) reported here excludes any ultrafast transfer from the 4 f spin angular momentum towards the orbital angular momentum in Gd. In addition, we rule out any ultrafast transfer from Co towards the Gd orbital momentum. Ultrafast demagnetization in CoTb For the Co 0.74 Tb 0.26 alloy the excited-state temperature is below T comp , thus leading to faster demagnetization rates for the RE ( τ therm =280±40 fs) as compared with other experiments where the excited-state temperature is in the vicinity of T C (refs 23 , 27 ). The pump-probe results measured at the Co L 2,3 and Tb M 4,5 edges are shown in Fig. 3a and transformed into ultrafast dynamics of S i ( t ) and L i ( t ) for Co and Tb as shown in Fig. 3b,c (red and black symbols). The normalized XMCD values at negative time delays match the XMCD magnitude recorded at the Co L 3 , Co L 2 , Tb M 5 and Tb M 4 edges during quantitative static XMCD measurements [27] . Applying the sum rules, we can extract the ultrafast dynamics of the spin and orbital momenta S i ( t ) (black circles) and L i ( t ) (red circles) for Co and for Tb. For Co and Gd we can neglect the magnetic dipole term T z ( t ) so that the spin momentum is then defined by S ( t )= S eff ( t ) [27] . For Tb, according to atomic calculations done by Teramura et al. [29] , we take T z / S =−0.08. We further correct the sum rule-extracted value S eff ( t ) by a value T z ( t ) [27] representing a time constant proportion of 8% of S ( t ). This assumption leads to an underestimation of 8% of S Tb ( t ) for t >0 assuming a virtual and complete quenching of T z ( t ) by the pump laser at t >0. The values at negative delays are normalized to the values measured at thermodynamic equilibrium [27] . The continuous lines correspond to the simulations of S i ( t ) (black line) and L i ( t ) (blue line; see Methods) while the green lines are the ratios between these numerical results. In Fig. 3b,c we observe an ultrafast quenching of S i ( t ) and L i ( t ) for Co and Tb. For each element, the thermalization times of S i ( t ) and L i ( t ) are identical (Co τ th =180±40 fs and Tb τ th =280±30 fs). Computing the ratio L i ( t )/ S i ( t ) reveals an ultrafast quenching for Co but for Tb any change is smaller than the error bars ( Fig. 3c , green symbols). 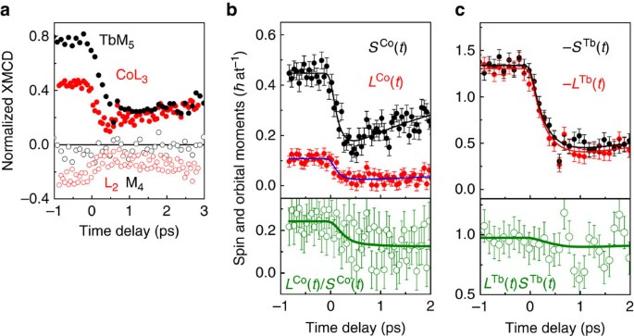Figure 3: Dynamics of spin and orbital momenta for Co and Tb in Co0,74Tb0,26. (a) Time-resolved XMCD at the Co L3(filled red circles), Co L2(empty red circles), Tb M5(filled black circles) and Tb M4edges (empty black circles) measured on a 15-nm Co0,74Tb0,26alloy film. The XMCD values at negative time delays match the XMCD magnitude recorded at the Co L3, Co L2, Tb M5and Tb M4edges during quantitative static XMCD measurements27. The pump fluence used during our experiment was adjusted to 12 mJ cm−2. (b) Ultrafast dynamics of the spin and orbital momentaSCo(t) (black circles) andLCo(t) (red circles) for Co extracted by applying the sum rules. The continuous lines are the simulations ofSCo(t) (black line) andLCo(t) (blue line; see Methods) with characteristic thermalization times ofτCotherm=180±40 fs for both momenta. The dynamics of the ratioLCo(t)/SCo(t) (green circle) shows that the orbital momentum decays more than the spin momentum during the ultrafast demagnetization. (c) Ultrafast dynamics of the spin and orbital momenta −STb(t) (black circles) and −LTb(t) (red circles) for Tb. The continuous lines are the simulations ofSTb(t) (black line) andLTb(t) (red line; see Methods) with characteristic thermalization times ofτTbtherm=280±40 fs for both momenta. The simulations ofLi(t) andSi(t) have been obtained using a nonlinear least square fitting procedure. The extracted error bar onτithermis the s.d., which is given as an output parameter of the fitting procedure. The error bars obtained forLi(t) andSi(t) as shown inbandcare given by the s.d. of the experimental data with respect to the fitting functions (see Methods). Figure 3: Dynamics of spin and orbital momenta for Co and Tb in Co 0,74 Tb 0,26 . ( a ) Time-resolved XMCD at the Co L 3 (filled red circles), Co L 2 (empty red circles), Tb M 5 (filled black circles) and Tb M 4 edges (empty black circles) measured on a 15-nm Co 0,74 Tb 0,26 alloy film. The XMCD values at negative time delays match the XMCD magnitude recorded at the Co L 3 , Co L 2 , Tb M 5 and Tb M 4 edges during quantitative static XMCD measurements [27] . The pump fluence used during our experiment was adjusted to 12 mJ cm −2 . ( b ) Ultrafast dynamics of the spin and orbital momenta S Co ( t ) (black circles) and L Co ( t ) (red circles) for Co extracted by applying the sum rules. The continuous lines are the simulations of S Co ( t ) (black line) and L Co ( t ) (blue line; see Methods) with characteristic thermalization times of τ Co therm =180±40 fs for both momenta. The dynamics of the ratio L Co ( t )/ S Co ( t ) (green circle) shows that the orbital momentum decays more than the spin momentum during the ultrafast demagnetization. ( c ) Ultrafast dynamics of the spin and orbital momenta − S Tb ( t ) (black circles) and − L Tb ( t ) (red circles) for Tb. The continuous lines are the simulations of S Tb ( t ) (black line) and L Tb ( t ) (red line; see Methods) with characteristic thermalization times of τ Tb therm =280±40 fs for both momenta. The simulations of L i ( t ) and S i ( t ) have been obtained using a nonlinear least square fitting procedure. The extracted error bar on τ i therm is the s.d., which is given as an output parameter of the fitting procedure. The error bars obtained for L i ( t ) and S i ( t ) as shown in b and c are given by the s.d. of the experimental data with respect to the fitting functions (see Methods). Full size image The ultrafast quenching of L Co ( t )/ S Co ( t ) in Co 0.8 Gd 0.2 and Co 0.74 Tb 0.26 leads to several conclusions. Interestingly, one notices that in this experiment we quenched L Co ( t )/ S Co ( t ) towards the value of 0.12, which is the value of hexagonal close packed Co (ref. 9 ). This reflects a transition from the highly anisotropic electronic distribution in Co–RE alloys towards the more isotropic distribution in hexagonal close packed structures. The quenching of L Co ( t )/ S Co ( t ) is in agreement with the model of ultrafast quenching of MCA proposed by Boeglin et al. [10] , in the framework of Bruno’s model [30] . This model predicts a direct relationship between the anisotropy of the orbital momentum and the magnetic anisotropy energy in 3 d TMs. In the case of 4 f -localized moments, the simple relationship given by Bruno [30] is no longer valid. Considering this limitation for RE 4 f moments, the ultrafast dynamics of L ( t )/ S ( t ) does not reflect the quenching of the MCA. However, the ultrafast dynamics of L Tb ( t )/ S Tb ( t ) observed in Fig. 3c (green line) is consistent with the fact that the 4 f moments are not directly pumped by the infrared laser but are exchange coupled with the laser pumped 3 d –5 d states, explaining a quasi-simultaneous demagnetization of L Tb ( t ) and S Tb ( t ), whereas the 3 d moments show an ultrafast quenching of L Co ( t )/ S Co ( t ). Considering the low infrared pump energy, we suggest that the exchange coupling between the 4 f and the pumped 5 d 3 d moments prevent large ultrafast quenching of the magnetocrystalline and dipolar anisotropy of the 4 f moments. It follows that under the given pump conditions, the proposed correction value of T z ( t ) as a constant proportion of S ( t ) is justified for Tb. Total angular momentum We calculate the angular momentum J i ( t )= L i ( t )+S i ( t ) by adding the element-resolved L i ( t ) and S i ( t ). We multiply J i ( t ) by the elemental concentration in the alloy for each i =Co, Gd or Tb in Co 0.8 Gd 0.2 ( Fig. 4a ) and Co 0.74 Tb 0.26 ( Fig. 4b ). All individual angular momenta J i ( t ) are quenched on laser excitation at t =0 ps. For each alloy, we then derive the total angular momentum J ( t )= J Co ( t )+ J Gd ( t ) ( Fig. 4a , blue open symbols) and J ( t )= J Co ( t )+ J Tb ( t ) ( Fig. 4b , blue open symbols). To account for the time dependence of T z ( t ) in Tb, we estimated the variation for J ( t ) to be ~0.020 ħ at −1 %, less than the given error bars of ±0.035 ħ at −1 %. In Co 0.8 Gd 0.2 , where the working temperature is close to but above T comp , we have J Co ≈− J Gd and the total angular momentum is mostly compensated. The remaining J ( t ) in CoGd is too small compared with the experimental noise level to reliably detect changes within the first few hundred of femtoseconds. The small negative values of J ( t ) observed for t >1 ps illustrates the non-equilibrium state of the system determined by the working temperature and pump conditions [27] . 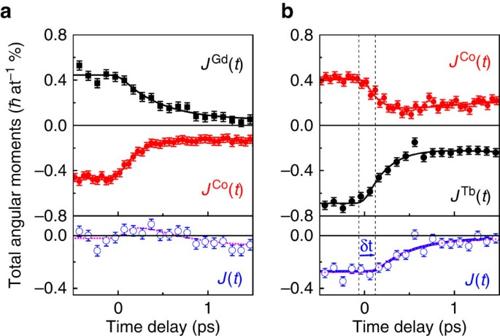Figure 4: Ultrafast dynamics of the individual and total angular momenta. (a) Angular momentaJCo(t) (red circles),JGd(t) (black circles) andJ(t)=JCo(t)+JGd(t) (blue circles) normalized by the composition (that is,JCo(t)=(LCo(t)+SCo(t)) × 0.80 andJGd(t)=(LGd(t)+SGd(t)) × 0.2) in the Co0,8Gd0.2film. The continuous lines are simulations ofJCo(t) (red line),JGd(t) (black line), whereas the magenta line is the sum of the two simulationsJCo(t) (red line) andJGd(t) (black line). (b) Angular momentaJCo(t) (red circles),JTb(t) (black circles) andJ(t)=JCo(t)+JTb(t) (blue circles) normalized by the composition (that is,JCo(t)=(LCo(t)+SCo(t)) × 0.74 andJTb(t)=(LTb(t)+STb(t)) × 0.26) measured in Co74Tb26alloy film. The continuous lines are simulations ofJCo(t) (red line),JTb(t) (black line) andJ(t) (blue line). The sum of both simulations (JCo(t)+JTb(t)—in magenta) cannot be distinguished from the simulation ofJ(t) (blue line). The loss of the total angular momentumJ(t) is delayed by δt=140±60 fs compared with the time at which the demagnetization of both sublattices starts. The simulations ofJi(t) andJ(t) have been obtained using a nonlinear least square fitting procedure. Error bars onJi(t) andJ(t) displayed inaandbcorrespond to the s.d. of experimental data with respect to the fitting functions (see Methods). Figure 4: Ultrafast dynamics of the individual and total angular momenta. ( a ) Angular momenta J Co ( t ) (red circles), J Gd ( t ) (black circles) and J ( t )= J Co ( t )+ J Gd ( t ) (blue circles) normalized by the composition (that is, J Co ( t )=( L Co ( t )+ S Co ( t )) × 0.80 and J Gd ( t )=( L Gd ( t )+ S Gd ( t )) × 0.2) in the Co 0,8 Gd 0.2 film. The continuous lines are simulations of J Co ( t ) (red line), J Gd ( t ) (black line), whereas the magenta line is the sum of the two simulations J Co ( t ) (red line) and J Gd ( t ) (black line). ( b ) Angular momenta J Co ( t ) (red circles), J Tb ( t ) (black circles) and J ( t )= J Co ( t )+ J Tb ( t ) (blue circles) normalized by the composition (that is, J Co ( t )=( L Co ( t )+ S Co ( t )) × 0.74 and J Tb ( t )=( L Tb ( t )+ S Tb ( t )) × 0.26) measured in Co 74 Tb 26 alloy film. The continuous lines are simulations of J Co ( t ) (red line), J Tb ( t ) (black line) and J ( t ) (blue line). The sum of both simulations ( J Co ( t )+ J Tb ( t )—in magenta) cannot be distinguished from the simulation of J ( t ) (blue line). The loss of the total angular momentum J ( t ) is delayed by δ t =140±60 fs compared with the time at which the demagnetization of both sublattices starts. The simulations of J i ( t ) and J ( t ) have been obtained using a nonlinear least square fitting procedure. Error bars on J i ( t ) and J ( t ) displayed in a and b correspond to the s.d. of experimental data with respect to the fitting functions (see Methods). Full size image For Co 0.74 Tb 0.26 where the working temperature is below T comp , we have J Co <− J Tb and a sizable value of J ( t )= J Co ( t )+ J Tb ( t ) is obtained that allows us to follow unambiguously the ultrafast dynamics of J ( t ). The validity of the determination of J ( t ) is supported by the limited error introduced by neglecting a virtual quenching of T z ( t ) at t >0. In such a case, we estimate that for J ( t ) we make an error of 0.025 ħ at −1 , well below the experimental error bars of 0.035 ħ at −1 given for the experimental values ( Fig. 4b ). Analysing the dynamics of J ( t ), we observe a loss of the total angular momentum J ( t ) towards an external bath until the value J ( t )≈0 is reached at t =1.5 ps. This dissipation happens with a characteristic time of 300±50 fs ( Fig. 4b ). At t =1.5 ps, the system is at quasi-equilibrium at a temperature close to T comp [27] and the value J ( t )=0 shows that the CoTb alloy is now magnetically compensated. The appealing feature is that the quenching of J ( t ) is delayed by δ t =140±60 fs, whereas both J Co ( t ) and J Tb ( t ) have already started to be quenched ( Fig. 4b ). The value δ t is estimated by performing simulations using a double exponential function for J ( t ) ( Fig. 4b , blue line; see Methods). In Fig. 4b we superpose the weighted sum of the two-fit functions obtained for J Co ( t ) and J Tb ( t ) as the magenta dotted line. The two-fit functions for J ( t ) agree perfectly. The delay of δ t =140±60 fs is attributed to an ultrafast transfer of angular momenta between the coupled Co and Tb sublattices. Compared with previous work by Medapalli et al. [31] and Graves et al. [24] , we provide quantitative time-resolved and element-selective angular momenta J i ( t ) in ferrimagnetic TM–RE alloys. Medapalli et al. [31] argued that a direct transfer of angular momentum occurs between the TM to the RE sublattices when the temperature of the sample is below the temperature of magnetic compensation. Although a model developed by Mentink et al. [22] supported their claim, no direct proof of such a mechanism has been provided so far. Graves et al. [24] discussed a non-local transfer of the angular momentum in FeCoGd films between chemically different nanograins. More recently, Wienholdt et al. [12] performed ab initio calculations using DFT to develop an orbital-resolved model for spin dynamics in RE–TM alloys. From their model, they concluded that the ferromagnetic-like state observed by Radu et al. [23] in FeCoGd is a consequence of ‘dissipationless spin dynamics’ during the first picoseconds after the excitation during which the energy and angular momentum is redistributed between the RE and TM elements. The experimental results presented here support this model. In our work we measure L i ( t ), S i ( t ) and J i ( t ) for each element and attribute the constant value of J ( t ) in Co 0.74 Tb 0.26 during the first 140 fs to the angular momentum flowing between J Co ( t ) and J Tb ( t ) ( Fig. 4b , blue symbols). This process is hidden in Co 0.8 Gd 0.2 because of the weak J ( t ). This mechanism allows an ultrafast and local demagnetization in both sublattices, whereas it conserves the total angular momentum J ( t ). We would like to point out that phonon- or defect-induced spin-flip scattering or superdiffusion of hot electrons would result in a decrease of J ( t ) if measured by XMCD. According to our analysis, these mechanisms do not show a major contribution up to 140±60 fs. After t =300 fs, the magnetization of Co reaches a minimum while the magnetization of Tb keeps decreasing, accompanied by a decrease of J ( t ). In this case, the transfer channel of angular momenta between sublattices is no more efficient and angular momentum is transferred from the Tb sublattice towards an external reservoir (phonons, hot electrons and so on). The transfer rate towards the external reservoir is now set by the transfer rate from the 4 f electrons, which is usually slower than that for the 3 d electrons in TM elements. We thus have clearly demonstrated that an efficient transfer channel for angular momenta exists in multisublattice ferrimagnetic alloys before any transfer to the external bath. This two-step transfer mechanism agrees perfectly with the theoretical calculations performed by Wienholdt et al. [12] . Furthermore, our results show that this transfer results from a direct exchange of angular momenta between Co and Tb as long as both sublattices are demagnetizing ( t <300 fs). In previous work by Radu et al. [23] , uncorrelated demagnetization between the two sublattices was detected in the sub-picosecond timescale. Going one step further and considering the quantitative angular momenta J i ( t ), we show here that the two sublattices are strongly linked between t =0 and 140±60 fs corresponding to the timescale of the exchange interaction [9] . To conclude, our findings demonstrate the local transfer of angular momenta between the two antiferromagnetically exchange-coupled sublattices. This transfer channel induces ultrafast demagnetization at the atomic scale, whereas the total angular momentum J ( t ) initially stays constant. In Co 0.74 Tb 0.26 we observed a delayed transfer of J ( t ) to an external bath. These results evidence a new ultrafast mechanism, determine the related timescale for angular momentum transfer during the demagnetization in ferrimagnetic systems and are supported by recent ab initio DFT calculations [12] . In addition, we have uncovered an ultrafast quenching of the L Co ( t )/ S Co ( t ) ratio in ferrimagnetic Co 0.8 Gd 0.2 and Co 0.74 Tb 0.26 alloys and attributed it to the ultrafast quenching of MCA in agreement with Bruno’s model and previous results in CoPd [10] , [30] . For the RE elements, a different behaviour is observed for L ( t )/ S ( t ) that could be linked to the localized character of the 4 f moments. Sample preparation and magnetic properties of the films Fifteen nanometres thick Co–RE alloys have been grown by magnetron sputtering on Si 3 N 4 membranes. Co-deposition with convergent Co and Gd (or Tb) flux was used to get amorphous Co 0.8 Gd 0.2 and Co 0.74 Tb 0.26 alloy films. The concentration in the films were optimized to obtain moderate saturation fields of 5 kOe or less, compatible with the magnet used in the time-resolved experiments. For Co 0.8 Gd 0.2 and Co 0.74 Tb 0.26 we have verified experimentally that at working temperatures the saturation fields are 4 and 3 kOe, respectively. Both alloys have been characterized by static XMCD [27] . As the samples were fully saturated by the external magnetic field of 5 kOe during the pump-probe experiments, we can define L z (resp. S z )= L (resp. S ) so that it follows that J i ( t )= L i ( t )+ S i ( t ) ( Fig. 4a , black and red symbols and Fig. 4b , black and red symbols) as the angular momentum of the element i (Co, Gd or Tb). The Co 0.8 Gd 0.2 and Co 0.74 Tb 0.26 films show magnetic compensation temperatures ( T comp ) at which both magnetizations of the Co and the RE sublattices compensate (resp. T comp =150 and 550 K) and Curie temperatures ( T C ) where the magnetic order is lost (resp. T C =450 and 650 K). The Co 74 Tb 26 alloy film presents an out-of-plane magnetic anisotropy, which is measured along the normal of the film plane. We emphasize that, in contrast to CoPd and Co 0.74 Tb 0.26 alloys [10] , [27] , Co 0.80 Gd 0.20 has no out-of-plane magnetic anisotropy. For this sample we performed our XMCD experiment at 30° from the normal of the film plane. In the case of Co 0.80 Gd 0.20 an in-plane uniaxial anisotropy may be induced during growth [32] . This point is confirmed by our recent results where static XMCD characterization was performed [27] . In both alloys we found large ratios L / S of 0.21–0.29 at the Co L 2,3 edges, whereas bulk Co shows a ratio of only 0.13. This is a strong indication for the presence of large MCA energies in all our Co–RE compounds. However, in our alloys, the quantitative value of the spin momentum (for instance, S Tb =1.35±0.2 at −1 ) is lower than expected from Hund’s rules ( S Tb =3 at −1 ) and is related to the structural disorder and finite temperature effects [27] . Time-resolved XMCD Time-resolved XMCD was performed at the femtoslicing beam line of the BESSY II synchrotron radiation source of the Helmholtz–Zentrum Berlin [7] , [10] . The magnetization dynamics have been measured by monitoring the transmission signal of circularly polarized X-rays, tuned to specific core-level absorption edges as a function of a pump-probe delay. The dynamic XMCD contrast is obtained by subtracting the gated signals obtained with and without pump beam. The energy was set to the different Co L 2,3 , Tb M 4,5 and Gd M 4,5 edges using the Bragg Fresnel reflection zone plate monochromator. The experiments have been performed with a pump-probe set-up where the short X-ray pulses are synchronized with a femtosecond pump laser working at 790 nm, 3 kHz repetition rate with pulses of 60 fs. The X-ray pulse duration of about 100 fs in the femtoslicing operation mode ensures a global time resolution of ~130 fs (see refs 7 , 10 for details). The pump fluences used during our experiments were adjusted to 8 mJ cm −2 for Co 0.8 Gd 0.2 and to 12 mJ cm −2 for Co 0.74 Tb 0.26 to reach large demagnetization magnitudes of about 60% at the Co L 3 edge without altering the sample properties (alloy concentration, atomic diffusion and large heating). Fitting procedure The physical quantities L i ( t ), S i ( t ) and J i ( t ) ( i =Co, Gd, Tb) were adjusted using the rate equation of the two-temperature model with two exponential functions (equation (1)): where G ( t ) is the Gaussian function defining the total time resolution of the experiment (130 fs), τ th and τ s−ph are the thermalization time and the relaxation time from the spin system to other systems (lattice, external bath), t 0 is the delay at which the temporal overlap of the pump and the probe is achieved and H ( t − t 0 ) is the Heaviside function ( H ( t − t 0 )=0 if t < t 0 and H ( t − t 0 )=1 if t > t 0 ) describing the energy transfer from the laser. The parameters C 0 , C 1 , t 0 and τ th in equation (1) were optimized to minimize independently the χ 2 factor for L i ( t ), S i ( t ) and J i ( t ) (equation (2)). where y is the rate equation, y j are the experimental data and σ j is the standard deviation (for j =1– n , and n is the number of data points). The minimization was performed via the Levenberg–Marquardt algorithm, based on a nonlinear least square procedure. The extracted error bars for τ th and t 0 correspond to the standard deviation (s.d. ), which is given as an output parameter of the fitting procedure. The error bars appearing in Figs 2b,c and 3b,c for L i ( t ) and S i ( t ) as well as on Fig. 4a,b for J i ( t ) correspond to the s.d. ( σ ) of experimental data with respect to the fitting functions that minimize the χ 2 factor. The amplitude of the error bars has been calculated according to equation (3): The final fitting parameters for J i ( t ) are compatible with the result of the sum of the two-fit functions obtained for L i ( t ) and S i ( t ). The total angular momentum for each alloy was obtained by performing the weighted sum J ( t )= J Co ( t )+ J Tb ( t ) according to the composition of the alloy. In Co 0.8 Gd 0.2 , the total angular momentum J Co ( t )+ J Gd ( t ) remains small and comparable to the noise level. For Co 0.74 Tb 0.26 , a sizable value of J ( t )= J Co ( t )+ J Tb ( t ) is obtained. In this case, we used the rate equation (1) to adjust J ( t ) (blue solid line in Fig. 4 ). In parallel, we plotted the weighted sum-of-the-fit functions obtained for J Co ( t ) and J Tb ( t ); (magenta dotted line in Fig. 4 ). The two-fit functions for J ( t ) agree perfectly for our parameters C o , C 1 , t 0 and τ th . The error bars given in Fig. 4a,b for J ( t ) correspond to the s.d. of the fitting function derived using equation (3). The results extracted from the rate equation lead to the following zero-time values: t 0 =0±40 fs for J Co ( t ) and J Tb ( t ) and t ′ 0 =140±40 fs for J ( t ), which allows us to define δ t =140±60 fs. The error bar for δ t has been derived as follows: Since the main source of uncertainty for δ t stems from the error bars of t 0 as extracted from the rate equation, we performed the simulations using a time axis for J Co ( t ) shifted by an amount of±40 fs with respect to J Tb ( t ). Doing so, we extracted the minimum and maximum delay times δ t for J ( t ) of 80 and 200 fs. These lower and upper limits define our error bar of 60 fs for the delais δ t =140 fs. How to cite this article: Bergeard, N. et al. Ultrafast angular momentum transfer in multisublattice ferrimagnets. Nat. Commun. 5:3466 doi: 10.1038/ncomms4466 (2014).